Organopolymer with dual chromophores and fast charge-transfer properties for sustainable photocatalysis Photocatalytic polymers offer an alternative to prevailing organometallics and nanomaterials, and they may benefit from polymer-mediated catalytic and material enhancements. MPC-1 , a polymer photoredox catalyst reported herein, exhibits enhanced catalytic activity arising from charge transfer states (CTSs) between its two chromophores. Oligomeric and polymeric MPC-1 preparations both promote efficient hydrodehalogenation of α -halocarbonyl compounds while exhibiting different solubility properties. The polymer is readily recovered by filtration. MPC-1 -coated vessels enable batch and flow photocatalysis, even with opaque reaction mixtures, via “backside irradiation.” Ultrafast transient absorption spectroscopy indicates a fast charge-transfer process within 20 ps of photoexcitation. Time-resolved photoluminescence measurements reveal an approximate 10 ns lifetime for bright valence states. Ultrafast measurements suggest a long CTS lifetime. Empirical catalytic activities of small-molecule models of MPC-1 subunits support the CTS hypothesis. Density functional theory (DFT) and time-dependent DFT calculations are in good agreement with experimental spectra, spectral peak assignment, and proposed underlying energetics. In spite of their comparative unsustainability, heterogeneous photocatalysts containing transition metal-based organometallic complexes and nanomaterials are well-precedented [1] , yet reports on heterogeneous organophotocatalysts are comparatively sparse [2] . Recently documented implementations include immobilization of dyes on various resin, silica, and polymer supports [3] , [4] , [5] , [6] , [7] , dye entrapment in polyethylene pellets [3] , soft gel dye entrapment [8] , immobilization of dyes onto metal-oxide films [9] , and incorporation into polymers as unconjugated pendant groups [10] . Although π -conjugated polymers are well-recognized with the 2000 Nobel Prize in Chemistry [11] , their direct application as macromolecular photocatalysts (MPCs) for organic synthesis is still nascent [12] . Carbon nitride systems have received substantial attention as inherently photocatalytic organopolymers, but their two-dimensional networks suffer from a lack of solution-processability [13] . The archetypal polymer of intrinsic microporosity, PIM-1 , was first reported in 2004 by Budd et al. [14] as a fluorescent yellow double-strand polymer prepared from a reaction of tetrafluoroterephthalonitrile ( 1 ) and a tetrahydroxyspirobiindane ( 2 ), yet to the best of our knowledge, its photoredox catalytic properties have not been reported. The precedent for the terephthalonitrile motif of PIM-1 in organophotoredox catalysis [2] , [15] , [16] suggests that PIM-1 and its analogs could be competent MPCs. Beyond the typical advantages of heterogenization (i.e., improved catalyst recyclability and product purity), organopolymer MPCs offer the possibility of leveraging a tunable macromolecular structure to enhance catalytic and material properties. A variety of reports have appeared documenting the modular tunability of PIM-1 properties through nitrile derivatization or co-incorporation of different monomers, especially for the purpose of changing the gas permeability of the resultant analog [17] , [18] . A PIM-1 analog, which proximally incorporates two distinct chromophores, separated by a flexible, conjugation-breaking spirocyclic comonomer, might be expected to provide catalytic enhancements in a manner analogous to organometallic systems. It is well-known that triplet metal-to-ligand charge-transfer ( 3 MLCT) states play a critical role in the photocatalysis of transition metal complexes [19] , [20] , [21] , [22] , [23] . Photoexcitation of electronic transitions from the ground-state to the singlet metal-to-ligand charge-transfer ( 1 MLCT) states is followed by the 1 MLCT→ 3 MLCT intersystem crossing (ISC) process. Transition metal complexes in the long-lived 3 MLCT states may act as either a reducing or an oxidizing agent. For organometallic photocatalysts, electron transfer takes place via an outer sphere process that involves electron tunneling between the catalyst and another molecule. In a dual-chromaphore PIM-1 analog, the charge-transfer states (CTSs) would instead arise from intramolecular transfer between separate chromophores, but these CTSs would likewise be associated with half-filled molecular orbitals and exhibit long lifetimes. Aside from potential enhancement of excited-state lifetime and catalyst–substrate redox processes, macromolecular structure provides additional means by which to adjust the overall catalytic process. In particular, catalyst solubility is tunable by monomer choice, feed ratio, and extent of polymerization. With appropriate solubility properties, organopolymer MPCs have the potential to be readily solution-processed into macroscopic structures such as thin-films, and it may be possible for the charge-transfer process to enable photoactivation when irradiating the film on the face not in contact with the reaction mixture (i.e., the face in contact with the wall of the vessel). Such a “backside irradiation” process could enable efficient photoactivation of systems suffering from poor light transmittance such as large-scale batch reactions and opaque reaction mixtures. Hydrodehalogenation is a mechanistically straightforward model reaction suitable for demonstration of photoredox catalyst efficacy and is also of general interest to the chemistry community. Thousands of halogenated natural products have been discovered in organisms ranging from bacteria to humans [24] , including chloramphenicol, one of the first three broad-spectrum antibiotics [25] , [26] . Conversely, halogens also feature in many persistent organic contaminants, which are not readily degraded by microbial systems [27] . Control of halogenation allows for modulation of the biological activity of chemical scaffolds, whether drug compounds or environmental contaminants [28] , [29] , [30] , and appreciation of the role of halogen binding in drug-target binding affinity increasingly influences drug discovery, development, and lead optimization [31] , [32] , [33] , [34] . Hydrodehalogenations have also long been utilized in synthetic strategy to remove halides that have served their purpose, e.g., for alkene protection [35] , iodocyclization [36] , or as a blocking group [37] , and similar opportunities for the beneficial application of this approach continue to appear. Traditional hydrodehalogenation methods, however, suffer from a number of problems with respect to toxicity, selectivity, recyclability, functional group tolerance, product purification, and operational simplicity. With recent advances in the scope of the three prevailing alternatives—ground-state organometallic catalysis [38] , metallophotoredox catalysis [39] , and organophotoredox catalysis [40] —the older methods should now be deprecated. Of these modern approaches, organophotoredox catalysis exhibits the best sustainability profile and is therefore an appropriate basis for a sustainability-oriented MPC system. We report herein the development of a dual-chromophore PIM-1 analog and its application as an organopolymer MPC to the mild hydrodehalogenation of α -halocarbonyl compounds. Benchmarking against common organophotoredox catalysts indicates that the MPC is more than five times as effective as its nearest competitor. The MPC can be efficiently recovered and reused, and it is effective when employed as a wall-coating in flow and batch reaction modes with backside irradiation, even with opaque reaction mixtures. The significance of the dual-chromophore system is supported by the catalytic activities of oligomeric compounds synthesized to model polymer substructures, as well as by ultrafast spectroscopic and computational studies. Preliminary investigation and optimization of conditions Our previous report on the synthesis of polyfluoro(hetero)aryl sulfones via micellar catalysis provided a wide variety of possible monomers for inclusion with 1 and 2 in the preparation of a PIM-1 analog [41] ; sulfone 3 was selected and the resultant MPC system was designated as MPC-1 (Fig. 1a ). We envisioned (and ultimately found) that sulfone 3 could imbue MPC-1 with suitable photophysical and solubility properties to function as an efficient and readily recoverable catalyst for hydrodehalogenation reactions (Fig. 1b ). In particular, we suspected that incorporation of 3 as a second chromophore subunit in the polymer would support the formation of long-lived CTSs during photoexcitation. We also anticipated that the solution-processability of MPC-1 would allow it to be applied as a coating to flow and batch reactors (Fig. 1c ). An initial preparation of the MPC-1 system (designated as MPC-1–0 ) was expeditiously synthesized in a one-pot adaptation of a previously reported polymerization procedure [17] starting from the precursors of 3 ; the targeted ratio of monomeric units of 1 , 2 , and 3 was 2:3:1. MPC-1–0 was encouragingly obtained as a bright yellow solid with a strong absorbance near 2.85 eV (435 nm), suggesting the possibility of visible-light catalysis with blue light-emitting diode (LED) irradiation (Supplementary Fig. 1 ). Although adequate for preliminary investigation, this preparation exhibited incomplete solubility in chloroform and under-incorporation of the sulfone monomeric unit; these deficiencies were attributed to incomplete sulfonylation and concomitant branching/cross-linking defects (see Supplementary Note 1 ). For initial reactivity screening, N -methyl-2-pyrrolidone (NMP) was selected as the reaction solvent given its aptitude for solubilization of structurally similar polymers [42] . 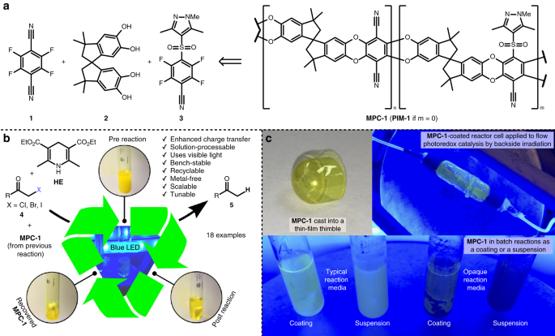Fig. 1 Structure and application of organopolymer photoredox catalystMPC-1.aConstituent monomers and representative structure ofMPC-1. The polymer is prepared by nucleophilic aromatic substitution, and chromophore subunits are randomly distributed.MPC-1is an analog ofPIM-1, which lacks sulfone monomer3.bα-Halocarbonyl compound hydrodehalogenation model reaction used to demonstrate the efficacy and advantages ofMPC-1.cProcessability ofMPC-1and its application. Preparations ofMPC-1have been cast into thin-film thimbles and applied as a coating to reaction vessels To our delight, NMP fully dissolved the polymer, and α -keto bromide 4a underwent hydrodehalogenation in the presence of i -Pr 2 NEt sacrificial reductant, 1 mol% MPC-1–0 (based on the molecular weight of the constitutional unit of an ideal regular polymer), and blue LED irradiation (Table 1 , entry 1). Control experiments confirm that the MPC-1 system catalyzed the transformation and that sacrificial reductant, blue LED irradiation, and oxygen-free atmosphere are all essential to catalysis (Supplementary Table 1 ). 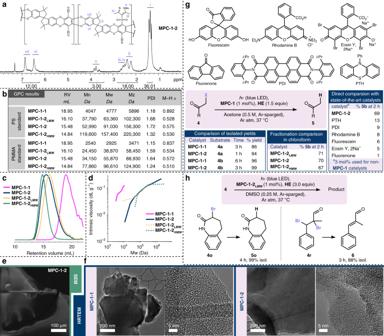Fig. 2 Characterization ofMPC-1preparations and assessment of catalytic activity.a1H NMR ofMPC-1–2with peak labels corresponding to proton locations.bTabulated gel permeation chromatography (GPC) results; PDI = polydispersity index.cGPC chromatograms.dMark–Houwink plots ofMPC-1preparations.eScanning electron microscopy (SEM) image of a sheet ofMPC-1–2.fHigh-resolution transmission electron microscopy (HRTEM) images ofMPC-1–1andMPC-1–2.gMPC-1activity studies: isolated yields of model substrates withMPC-1–1andMPC-1–2, comparison ofMPC-1–2fractionations in chloroform, and comparison with benchmarking catalysts; PTH = 10-phenylphenothiazine; PDI =N,N-bis(2,6-diisopropylphenyl)perylene-3,4,9,10-bis(dicarboximide).hMPC-1–2efficacy with hydrodehalogenation of a less reactive substrate and deprotection of a brominated ene-aldehyde. Source data are provided as a Source Data file Screening catalyst loading confirmed that 1 mol% MPC-1–0 was suitable for preliminary optimization (Supplementary Table 2 ). Solvent screening revealed a clear correlation between reaction efficiency and solvent polarity index [43] (Table 1 , entries 1–6), suggesting the reaction pathway involves excited-state charge separation, which is more effectively stabilized by more polar solvents [44] . NMP was the only solvent capable of fully dissolving the polymer, but the ability of the solvent to dissolve MPC-1–0 (which was used as a finely ground powder) was of limited importance, indicating that the catalyst worked well in both homogenous and heterogeneous states. Indeed, although NMP was the most effective solvent, dimethyl sulfoxide (DMSO) was nearly as competent and is a far greener choice [45] . Water is the greenest solvent, has the highest polarity index, and appeared competent with 41% conversion after 1 h, but the poor solubility of 4a in water led to clumping of the substrate into a solid mass on the spin-vane, preventing the reaction from going to completion. An aqueous solution of anionic surfactant sodium dodecyl sulfate (SDS, entry 8) likewise permitted partial reaction progress, but the reaction mixture eventually developed clumping and opacity that prevented reaction completion. Isolated yields of reactions run with i -Pr 2 NEt were consistently poor (ca. 40%) due to side reactions, but switching the reductant to Hantzsch ester ( HE ) dramatically increased reaction rate and yield (entry 9). Following optimization of HE loading, acetone was deemed sufficiently competent and was selected as a green and easily distillable reaction medium [45] . With the final optimized conditions, dehalogenated product 5a was successfully obtained in 92% isolated yield after 3 h in acetone with 1.5 equiv HE and 1 mol% MPC-1–0 (entry 10). Full optimization results are provided in Supplementary Tables 2 – 9 . Fig. 1 Structure and application of organopolymer photoredox catalyst MPC-1 . a Constituent monomers and representative structure of MPC-1 . The polymer is prepared by nucleophilic aromatic substitution, and chromophore subunits are randomly distributed. MPC-1 is an analog of PIM-1 , which lacks sulfone monomer 3 . b α -Halocarbonyl compound hydrodehalogenation model reaction used to demonstrate the efficacy and advantages of MPC-1 . c Processability of MPC-1 and its application. Preparations of MPC-1 have been cast into thin-film thimbles and applied as a coating to reaction vessels Full size image Table 1 Optimization of reaction conditions. Full size table Reaction scope and scalability with oligomeric MPC-1–1 A new procedure was developed to produce oligomeric MPC-1 , designated as MPC-1–1 , while avoiding the defects associated with the one-pot procedure used for MPC-1–0 . Polymerization was conducted in 3 wt% aqueous PS-750-M surfactant using separately synthesized sulfone 3 ; the feed ratio of monomers 1 , 2 , and 3 was 2:3:1. PS-750-M was designed to mimic toxic polar aprotic solvents such as DMF [46] , which had been employed in the synthesis of MPC-1–0 . Typically, PIM-1 analogs are synthesized under anhydrous conditions [17] . By intentionally using an aqueous system, it was possible to severely restrict polymer chain length through the facile termination of chain growth by hydroxide replacement of fluorine; the micelles assisted in protecting the aromatic fluorides until polymer size was sufficiently large to precipitate out of the solution. MPC-1–1 successfully obtained as an opaque yellow solid that was readily soluble in acetone. Nuclear magnetic resonance (NMR) and gel permeation chromatography (GPC) measurements suggested that the average chain length of MPC-1–1 was sufficiently long to incorporate 4–7 chromophore subunits (i.e., monomer units of 1 or 3 ); although successful in producing oligomeric chains, this method was still susceptible to branching defects and appeared to under-incorporate the terephthalonitrile monomeric unit (see Supplementary Note 1 ). Using MPC-1–1 under the optimized reaction conditions afforded 5a in 86% isolated yield after 3 h, indicating that the activity of the oligomeric preparation was slightly inferior to MPC-1–0 . It was initially suspected that the catalytic activity of MPC-1 preparations would improve with higher degrees of polymerization; because MPC-1–1 represents a non-arbitrary lower limit in this regard, it was used to establish well-defined baseline substrate scope results. Longer-chain MPC-1 preparations indeed performed better, but the origin of this improvement turned out to be more complicated (vide infra). A wide-range of α -halocarbonyl compounds were amenable to hydrodehalogenation under the established conditions. As suggested by the chemoselectivity in the reaction used for optimization, aryl halides (which exhibit a larger reduction potential) were unaffected by the reaction conditions (Table 2 , 4a–h ). Aside from ketones ( 4a–n ), alkyl aryl ethers ( 4e ), aryl nitro groups ( 4 l ), amides ( 4o ), and esters ( 4p ) were also well tolerated. α -Keto chlorides, bromides, and iodides were reduced with rates that increased with decreasing magnitude of substrate reduction potential ( 4b–d ). With a sufficient quantity of reductant, geminal bromides were both reduced ( 4 m ); when only 1 equiv reductant was used, a roughly equal mixture of acetophenone and 2-bromoacetophenone products was observed. Greater steric bulk around the halide did not prevent reduction, but rate was affected in accordance with the effect of the geminal alkyl substituents on the stabilization of a radical intermediate ( 4h–j ). In addition to α -aryl keto carbonyl systems ( 4a–m ), reduction was successful with strained aliphatic ( 4n ) and heteroaromatic ( 4q ) ketones, as well as for α -amide ( 4o ) and α -ester ( 4p ) systems. The reactions were generally clean, affording only oxidized HE and the desired product. Table 2 α-Halocarbonyl compound hydrodehalogenation scope and scalability with MPC-1–1 a Full size table Scalability and catalyst recovery were demonstrated with the gram-scale hydrodehalogenation of 4b (Table 2 ). With a lowered catalyst loading, i.e., 0.2 mol%, product 5b was afforded in 99% isolated yield after 24 h. In addition to the lower catalyst loading, the longer reaction time is partly attributable to the change in reaction vessel and the resultant decrease in flux of irradiation. The reaction was worked up by removing acetone under reduced pressure and extracting the product with 1:14 ethyl acetate/hexanes, a solvent system in which MPC-1–1 was insoluble. To liberate product entrapped in the polymeric phase, ethyl acetate was admixed first before precipitating the polymer back out with the addition of hexanes. A preliminary recycle study using this extraction technique confirmed that the catalyst remained active in subsequent cycles, but buildup of residual Hantzsch pyridine caused the reaction rate to decrease (see Supplementary Method 1 ). This limitation to recyclability was overcome with the development of a longer-chain MPC-1 preparation, MPC-1–2 , which was fully recyclable and retained its catalytic efficiency over multiple recycles (vide infra). Synthesis and evaluation of polymeric MPC-1–2 Rigorous polymerization conditions were devised to yield long chains with limited cross-linking defects. Monomer 1 was purified by sublimation, monomer 2 was recrystallized from methanol/water, monomer 3 was purified by column chromatography, and potassium carbonate was dried in a vacuum oven at 200 °C overnight prior to use. The polymerization was conducted in a thick-walled Schlenk tube under argon atmosphere at 90 °C in dry N,N -dimethylacetamide (DMAc). Activated 3 Å molecular sieves were included in the reaction mixture to scavenge moisture. Upon reaction completion, the reaction mixture was extracted with chloroform and the product was precipitated out with the addition of methanol. Thus, resultant polymer preparation MPC-1–2 was obtained as a translucent yellow solid. To assess the significance of different polymer chain lengths within MPC-1–2 , which had a moderate polydispersity index, a portion of the material was further processed by thrice reprecipitating from chloroform with methanol such that the polymer mass in the precipitate was approximately equal to the polymer mass in the combined supernatant layers; the higher molecular weight fractionation from the precipitate is designated as MPC-1–2 HMW , and the lower molecular weight fractionation from the supernatant layers is designated as MPC-1–2 LMW . MPC-1–2 1 H NMR integrations were in good agreement with the 2:3:1 feed ratio of 1 , 2 , and 3 (Fig. 2a ): the alkyl methyl signals from 2 (labeled as i) integrated to 36; the methylene signals of 2 (ii) and the overlapping aryl methyl signals of 3 (iii and iv) integrated to 18; the N -methyl signals of 3 (v) integrated to 3; and the aromatic signals of 2 (labeled as vi and vii) integrated to 12. Sulfone 3 was moderately over-incorporated in fractionation MPC-1–2 LMW (3:1.14 ratio of 2 and 3 ) and under-incorporated in MPC-1–2 HMW (3:0.88 ratio of 2 and 3 ); this variation suggests either that the fractionation method is partly affected by the solubility of randomly incorporated constituent monomers, or that shorter chains tend to incorporate greater amounts of 3 (see Supplementary Note 1 ). Acetone admixed with MPC-1–2 LMW developed coloration but did not completely dissolve the solid, whereas acetone admixed with MPC-1–2 HMW remained colorless, suggesting that an acetone-soluble component in MPC-1–2 had been at least mostly confined to the MPC-1–2 LMW fractionation. Fig. 2 Characterization of MPC-1 preparations and assessment of catalytic activity. a 1 H NMR of MPC-1–2 with peak labels corresponding to proton locations. b Tabulated gel permeation chromatography (GPC) results; PDI = polydispersity index. c GPC chromatograms. d Mark–Houwink plots of MPC-1 preparations. e Scanning electron microscopy (SEM) image of a sheet of MPC-1–2 . f High-resolution transmission electron microscopy (HRTEM) images of MPC-1–1 and MPC-1–2 . g MPC-1 activity studies: isolated yields of model substrates with MPC-1–1 and MPC-1–2 , comparison of MPC-1–2 fractionations in chloroform, and comparison with benchmarking catalysts; PTH = 10-phenylphenothiazine; PDI = N , N -bis(2,6-diisopropylphenyl)perylene-3,4,9,10-bis(dicarboximide). h MPC-1–2 efficacy with hydrodehalogenation of a less reactive substrate and deprotection of a brominated ene-aldehyde. Source data are provided as a Source Data file Full size image GPC results were obtained using an Omnisec GPC from Malvern, which was equipped with four on-line detectors: a dual-angle light scattering detector, an ultraviolet (UV) detector, a refractive index detector, and a viscosity detector (Fig. 2b ). In the chromatogram (Fig. 2c ), the refractive index peak of MPC-1–2 is situated between MPC-1–2 LMW and MPC-1–2 HMW while its distribution covered the range of both components, which was consistent with the tabulated results. Minor peaks indicating the existence of oligomers were observed at retention volume >19 mL for MPC-1–2 and its fractionations. All four samples were fully soluble in the tetrahydrofuran eluent, and Mark–Houwink plots were also constructed to assess their structures (Fig. 2d ). The curves of MPC-1–2 and its fractionations overlapped with each other at a wide-range, which implied a similar Mark–Houwink exponent (M–H α ) and the same branching degree with the different polymer compositions. Fourier-transform infrared spectroscopy showed that all monomers were incorporated into the derivative polymers, and MPC-1–2 lacked the hydroxyl stretches present in MPC-1–1 (Supplementary Fig. 2 ). Both MPC-1–1 and MPC-1–2 exhibited high thermal stability when subjected to thermogravimetric analysis (TGA) and differential scanning calorimetry (DSC), which showed very little change up to 200 °C, followed by a gradual loss of mass until 450 °C (Supplementary Fig. 3 ). A sheet of MPC-1–2 was subjected to scanning electron microscopy (SEM); the sheet was observed to be regular and smooth (Fig. 2e ). High-resolution transmission electron microscopy (HRTEM) imaging of MPC-1–1 and MPC-1–2 showed that MPC-1–2 had a more regular macrostructure consisting of large layers of stacked sheets while MPC-1–1 had smaller planes of sheets with smaller and rounder edges (Fig. 2f ). At high magnification, both samples were seen to exhibit a similar porous structure. Inductively coupled plasma mass spectrometry (ICP-MS) confirmed the absence of iridium and ruthenium traces, which otherwise might be responsible for observed photocatalytic activity. Having made and characterized a variety of MPC-1 preparations, we sought to assess their catalytic activities and generalize the results by benchmarking against well-known organophotoredox catalysts (Fig. 2g ). Higher isolated yields for hydrodehalogenation of bromide 4a and chloride 4b were obtained in less time with MPC-1–2 compared to MPC-1–1 . Unsurprisingly, MPC-1–2 exhibited improved catalytic activity in acetone when used as a fine powder instead of larger pieces, which would be expected to remain undissolved and thereby exclude interior active units from participating in catalysis. Accordingly, to better exclude influence of active unit entrapment in the interior of undissolved solid, the catalytic activities of MPC-1–2 and its fractionations were compared with the hydrodehalogenation of 4b in chloroform, a reaction medium in which all were fully soluble; observed activities were nearly the same. MPC-1–2 was benchmarked against six common organophotoredox catalysts [2] using the same model reaction in acetone. MPC-1–2 proved to be the best by far, catalyzing more than five times as much product formation as its nearest competitor in the timeframe of the experiment. Leveraging the improved catalytic activity of MPC-1–2 , difficult substrate 4o was hydrodehalogenated with significant improvements to reaction rate and yield, and a vicinal dibromide was efficiently converted into the corresponding alkene (Fig. 2h ). Recyclability of MPC-1–2 The altered solubility properties of MPC-1–2 appeared promising for improved recycling techniques. A batch reaction recycle study was conducted using MPC-1–2 LMW for the hydrodehalogenation of 4b under standard conditions (Fig. 3a ). The partial solubility of MPC-1–2 LMW in the reaction medium was readily overcome upon reaction completion with the addition of methanol, whereupon the suspension was passed through a fritted glass funnel to separate the catalyst from the rest of the reaction mixture. The catalyst could then be returned to the reaction vessel as a solid or through solution processing to pass it through the frit; these two approaches worked equally well. Six reaction cycles were conducted in this manner without appreciable decrease in catalyst activity. The complete acetone solubility and limited methanol solubility of MPC-1–1 made this approach infeasible for the oligomeric system. Fig. 3 Batch and flow recyclability of MPC-1–2 . a Recycle study with MPC-1–2 LMW . Each recycle, additional 4b (0.25 mmol) and HE (0.375 mmol) were added to the recovered MPC-1–2 LMW catalyst (1 mol%, approximated as 1529 g mol −1 ) originating from the zeroth cycle; the reaction vessel was sealed, thrice evacuated/argon-backfilled, filled with 0.5 mL argon-sparged acetone, then stirred at 37 °C under blue LED irradiation for 3 h. MPC-1–2 LMW was recovered by diluting the reaction mixture with 0.5 mL methanol and passing it through a fritted glass funnel; the catalyst was then returned to the reaction vessel by spatula or by passing it through the frit with dichloromethane. b Flow chemistry with MPC-1–2 HMW as a thin-film coating. Reaction conditions: 4b (0.7 mmol, placed in the reservoir), HE (1.05 mmol, placed in the reactor cell), acetonitrile (3.5 mL, argon-sparged), argon atmosphere, peristaltic circulation through an MPC-1–2 HMW -coated (2.5 mol%) reactor cell under blue LED irradiation, 37 °C, 26 h Full size image To further demonstrate the unique possibilities afforded by an innately photocatalytic solution-processable polymer, a new approach to catalyst recycling under flow conditions was envisioned wherein the photocatalytic polymer would be coated on the walls of a flow cell. The reaction solvent would be selected so as not to dissolve the coating. Following a post-reaction rinse, the flow cell could then be reused in subsequent reactions. Although a precedent exists for flow cells containing heterogenized photoredox catalyst immobilized by polymer support or sol–gel techniques [47] , to the best of our knowledge the wall-coating of a transparent and inherently photocatalytic polymer on the walls of a flow cell has not yet been reported. We fashioned a prototype large-volume flow cell to accommodate the poorly soluble reductant and coated its walls by dissolving MPC-1–2 HMW in dichloromethane, which was allowed to evaporate as the cell was rotated. The flow cell was loaded with HE and an acetonitrile solution of 4b was peristaltically circulated from a reservoir through the cell, which was subjected to blue LED irradiation (Fig. 3b ). The polymer coating was retained on the walls of the flow cell throughout the course of the reaction, and after 26 h the reactor loop was drained into the reservoir and the product was isolated in 83% yield, confirming the viability of the concept. It is noteworthy that MPC-1–2 HMW was required for retention of the coating; unfractionated MPC-1–2 was gradually stripped from the walls under reaction conditions. Mechanistic studies and assessment of backside irradiation A series of control studies were conducted with halide 4b , which confirmed that hydrodehalogenation product 5b only formed in the simultaneous presence of MPC-1 , HE , and blue LED irradiation; no conversion was observed when one or more of these components was omitted (Supplementary Table 1 ). Subsequently, the ground-state redox potentials of the control reaction components were determined experimentally by cyclic voltammetry, and the excited-state redox potentials of the catalyst were estimated using the polymer emission wavelength. On the basis of this information, a plausible mechanism is proposed (Fig. 4a ). The need for the sacrificial reductant indicates that, as is often the case with the monomeric analog p -dicyanobenzene, MPC-1 is operating as an excited-state oxidant [2] , and the reactivity-determining potential is that of the reduced form, MPC-1 •– ( E ox = –1.42 V vs. SCE). Thus, following photoexcitation, MPC-1* ( E red = 1.01 V vs. SCE) is reductively quenched through single electron transfer (SET) from reductant HE ( E ox = 0.89 V vs. SCE). Subsequently, SET from MPC-1 •– to halide 4b ( E red = –1.24 V vs. SCE) leads to homolytic cleavage of the carbon–halogen bond. The resultant alkyl radical is then converted to the product by forming a bond with a methylene hydrogen from HE •+ as it establishes aromaticity to form Hantzsch pyridine. Fig. 4 Investigation of mechanism and viability of backside irradiation. a Proposed mechanism. b Activity screening of polymer subunit models; all models were prepared as mixtures of isomers. c Illustration of backside irradiation. d Results of charcoal occlusion study for coatings and suspensions of MPC-1–2 HMW . Source data are provided as a Source Data file Full size image Well-defined models of MPC-1 substructures 7 – 11 were synthesized to better elucidate the effects of chain formation and dual chromophores (Fig. 4b ). The activity of the models was assessed with the same reaction conditions used for the benchmarking studies (Fig. 2g ); the catalyst loading was adjusted to maintain a constant amount of active chromophore units across experiments. Catalyst model 7 , which contained one sulfone chromophore, was inferior to all other models with only 27% yield after 2 h. The other single chromophore model, 8 , which contained the terephthalonitrile motif, was highly active, providing 99% product in the same timeframe. As the chain length was increased with models 9 and 10 , the yield decreased (97% and 84%, respectively); this observation was in agreement with the expectation that yield would decrease with decreasing molecular concentration of catalyst even though active unit loading was held constant. However, when using catalyst model 11 , which replaced the middle terephthalonitrile unit in 10 with the less active sulfone chromophore, the activity was superior to even single terephthalonitrile model 8 ; this improved activity in spite of lower molecular catalyst concentration and partial use of the less effective sulfone chromophore is in agreement with the charge-transfer state hypothesis. An additional experiment using a 1:2 ratio of models 7 and 8 afforded only 93% yield, indicating that the dual-chromophore activity enhancements are only present when the two-chromophore types are incorporated into the same molecule. To further demonstrate the impact of this catalyst, backside irradiation technology was explored as a proof-of-concept (Fig. 4c ). This technology could prove useful for reaction mixtures with low light transmittance. Four reactions were set-up in parallel; two vessels contained a wall-coating of MPC-1–2 HMW , and two contained the catalyst as a suspension; in one of each of the vessel sets, the reaction mixture was made opaque with the inclusion of charcoal (Fig. 1c , Fig. 4d ). The hydrodehalogenation of 4b was more efficient with a wall-coating than with a suspension, even with the inclusion of charcoal, supporting that the backside irradiation process played a role (Fig. 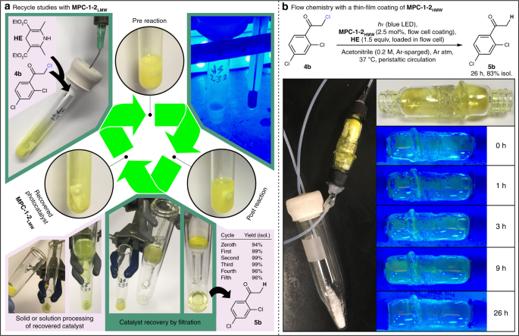Fig. 3 Batch and flow recyclability ofMPC-1–2. a Recycle study withMPC-1–2LMW. Each recycle, additional4b(0.25 mmol) and HE (0.375 mmol) were added to the recoveredMPC-1–2LMWcatalyst (1 mol%, approximated as 1529 g mol−1) originating from the zeroth cycle; the reaction vessel was sealed, thrice evacuated/argon-backfilled, filled with 0.5 mL argon-sparged acetone, then stirred at 37 °C under blue LED irradiation for 3 h.MPC-1–2LMWwas recovered by diluting the reaction mixture with 0.5 mL methanol and passing it through a fritted glass funnel; the catalyst was then returned to the reaction vessel by spatula or by passing it through the frit with dichloromethane.bFlow chemistry withMPC-1–2HMWas a thin-film coating. Reaction conditions:4b(0.7 mmol, placed in the reservoir), HE (1.05 mmol, placed in the reactor cell), acetonitrile (3.5 mL, argon-sparged), argon atmosphere, peristaltic circulation through anMPC-1–2HMW-coated (2.5 mol%) reactor cell under blue LED irradiation, 37 °C, 26 h 4c ). Likewise, coated vessels are not affected by the occlusion of light caused by undissolved HE : the trend in conversion over time for coated reaction vessels lacks the inflection point observed for vessels with catalyst suspension; this inflection point is attributable to opaque, poorly soluble HE being sufficiently converted to Hantzsch pyridine to allow for improved light transmittance. Quantum chemical calculations To aid in understanding the energetics and electronic structure of the MPCs, density functional theory (DFT) and time-dependent (TD-)DFT calculations were performed at the B3LYP/6–31 G(d) level of theory, utilizing the Frenkel-Davydov exciton model to interpret the results [48] , [49] , [50] , [51] , [52] (see Supplementary Note 2 and Supplementary Fig. 4 ). The investigations were carried out on a hypothetical heterodimer subunit, D XY , as well as the isolated chromophores, X and Y , present in MPC-1 chains (Fig. 5a ). 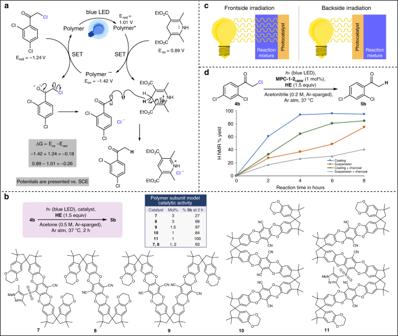Fig. 4 Investigation of mechanism and viability of backside irradiation.aProposed mechanism.bActivity screening of polymer subunit models; all models were prepared as mixtures of isomers.cIllustration of backside irradiation.dResults of charcoal occlusion study for coatings and suspensions ofMPC-1–2HMW. Source data are provided as a Source Data file All DFT/TD-DFT calculations were performed using Gaussian 16 Rev. A.03 [53] . The polarizable continuum model (PCM) was employed to simulate the solvent effect of chloroform. 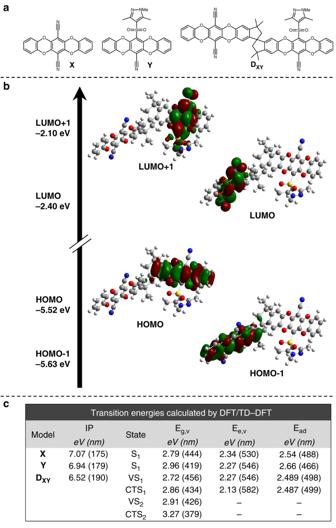Fig. 5 Overview of the density functional theory (DFT)/time-dependent (TD-)DFTresults.aStructures of chromophore modelsX,Y, and heterodimerDXYinvestigated by DFT/TD-DFT calculations.bFrontier molecular orbitals of the investigatedDXYheterodimer with DFT-calculated orbital energies labeled on the left.cSummary of transition energies resulting from DFT/TD-DFT calculations. IP = ionization potential,Eg,v= vertical excitation energy at ground-state equilibrium geometry,Ee,v= vertical excitation energy at excited-state equilibrium geometry,Ead= adiabatic excitation energy. Source data are provided as a Source Data file Figure 5b depicts frontier molecular orbitals of the D XY heterodimer model and their energies predicted by DFT. Fig. 5 Overview of the density functional theory (DFT)/time-dependent (TD-)DFTresults. a Structures of chromophore models X , Y , and heterodimer D XY investigated by DFT/TD-DFT calculations. b Frontier molecular orbitals of the investigated D XY heterodimer with DFT-calculated orbital energies labeled on the left. c Summary of transition energies resulting from DFT/TD-DFT calculations. IP = ionization potential, E g,v = vertical excitation energy at ground-state equilibrium geometry, E e,v = vertical excitation energy at excited-state equilibrium geometry, E ad = adiabatic excitation energy. Source data are provided as a Source Data file Full size image TD-DFT calculations were carried out to predict the transition energies of the first few excited states of X , Y , and D XY at ground-state equilibrium geometry (cartesian coordinates are listed in Supplementary Note 3 ). After characterizing the states of interest, geometry optimization of the first excited states (S 1 ) of both X - and Y -chromophores and the first valence state (VS 1 ), as well as the first charge-transfer state (CTS 1 ) of the D XY heterodimer were performed. Geometry optimization of the second valence state (VS 2 ) and the second charge-transfer states (CTS 2 ) of D XY converged to the VS 1 and CTS 1 state, respectively. Frontier molecular orbitals and transition energies resulting from these calculations are briefly summarized in Fig. 5b, c , respectively (further details are provided in Supplementary Note 4 , Supplementary Figs. 5 and 6 , and Supplementary Table 10 ). The observation that the vertical excitation energy of VS 1 is smaller than that of CTS 1 at the ground-state geometry ( E g,v (VS 1 ) < E g,v (CTS 1 )), while the adiabatic excitation energy of VS 1 is larger than that of CTS 1 ( E ad (VS 1 ) > E ad (CTS 1 )), suggests the existence of a conical intersection (CI) between these two states. However, due to the size of the heterodimer model, no multiconfiguration calculations were attempted to locate the CI. Steady-state absorption and photoluminescence spectra The UV–visible(Vis) absorption and photoluminescence (PL) spectra of MPC-1–1 and MPC-1–2 are presented in Fig. 6a . Both absorption spectra consist of a relatively broad peak approximately centered at 2.9 eV (428 nm) and a stronger peak located around 4.3 eV (288 nm). The PL spectra are dominated by a peak centered at 2.54 eV (488 nm) with a long tail extending into the red region (~ 2.0 eV, ~ 620 nm). Fig. 6 Overview of measured absorption and photoluminescence spectra for MPC-1 systems and time-dependent (TD)-DFT-predicted absorption spectra. a Overlay of normalized ultraviolet (UV)–visible(Vis) absorption (Abs) and photoluminescence (PL) spectra of the investigated MPC-1–1 (black) and MPC-1–2 (red). PL excitation energy, hν ex = 2.95 eV ( λ ex = 420 nm). b Overlay of normalized absorption spectra (solid curves) of X - (green) and Y - (magenta) chromophores, and D XY heterodimer (blue) simulated using TD-DFT-calculated transition energies and intensities at the ground-state equilibrium geometry. Corresponding transitions are shown as an overlaid stick plot with matching colors. Simulated spectra were generated using a Gaussian lineshape of a width ( σ ) = 0.15 eV. 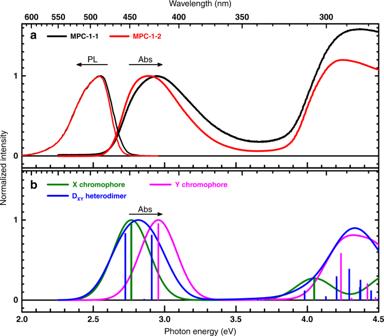Fig. 6 Overview of measured absorption and photoluminescence spectra forMPC-1systems and time-dependent (TD)-DFT-predicted absorption spectra.aOverlay of normalized ultraviolet (UV)–visible(Vis) absorption (Abs) and photoluminescence (PL) spectra of the investigatedMPC-1–1(black) andMPC-1–2(red). PL excitation energy,hνex= 2.95 eV (λex= 420 nm).bOverlay of normalized absorption spectra (solid curves) ofX- (green) andY- (magenta) chromophores, andDXYheterodimer (blue) simulated using TD-DFT-calculated transition energies and intensities at the ground-state equilibrium geometry. Corresponding transitions are shown as an overlaid stick plot with matching colors. Simulated spectra were generated using a Gaussian lineshape of a width (σ) = 0.15 eV. Source data are provided as a Source Data file 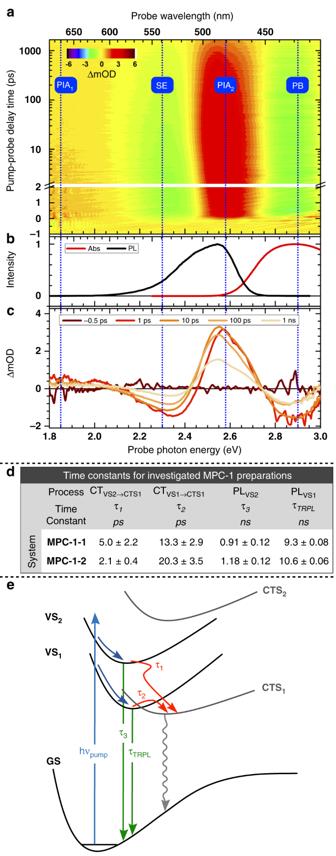Fig. 7 Overview of transient absorption (TA) results and electronic model.aPseudo-color map representing the TA spectra ofMPC-1–2.bUltraviolet (UV)–visible (Vis) absorption (Abs) and PL spectra ofMPC-1–2.cAbsorption difference spectral lines at various delays showing the position and evolution of the four features observed in the TA spectra.dTime constants of processes of interest extracted from fitting TA (τ1–τ3) and TRPL (τTRPL) kinetics; CTVS2→CTS1, CTVS1→CTS1, PLVS2, and PLVS1indicate the` physical process associated with each time constant, respectively. Error bars represent the standard error at 1σ.eSchematic of potential energy curves of the lowest electronic states of the heterodimer,DXY. Source data are provided as a Source Data file Source data are provided as a Source Data file Full size image Figure 6b shows the predicted absorption spectra of X and Y chromophores and the heterodimer D XY . The simualted spectrum of the heterodimer is in good agreement with the experimantal spectra of both MPC-1–1 and MPC-1–2 . The lowest-energy peak at ~ 2.9 eV (428 nm) is assigned to the VS 1 \(\leftarrow\) GS and VS 2 \(\leftarrow\) GS transitions, predicted by TD-DFT calculations for the heterodimer to be at 2.72 eV (456 nm) and 2.91 eV (426 nm), respectively. The higher-energy peak is also predicted by TD-DFT calculations. Figure 6b also demonstrates that most bright states of the heterodimer are closely associated with those of the isolated chromophores X and Y . This observation implies a possibility of decomposing the experimental absorption and PL spectra of both MPC-1–1 and MPC-1–2 . Decomposition was carried out using two Gaussian lineshapes, corresponding to contributions from X and Y chromophores. Assignment of the decomposed electronic transitions is aided by the TD-DFT-predicted transition energies (Fig. 5c ). Briefly, the higher-energy absorption band, and the lower-energy emission band are assigned to electronic transitions localized at the Y chromophore, while the lower-energy absorption band and the higher-energy emission band are assigned to transitions localized at the X chromophore. The resulting central transitions and Stokes shifts from the decomposition of absorption and PL spectra are in good agreement with the energetics of X and Y chromophores predicted by TD-DFT (results are summarized in Supplementary Note 5 , Supplementary Fig. 7 , and Supplementary Table 11 ). The slight blue shift of the MPC-1–1 absorption peak from that of MPC-1–2 is likely due to the difference in their chromomphoric composition as discussed in Supplementary Note 1 . Femtosecond transient absorption spectroscopy Transient absorption (TA) spectra of both MPC-1–1 and MPC-1–2 shared similar main features (Fig. 7a and Supplementary Fig. 8 ). Following photoexcitation with a 3.2 eV (388 nm) laser pulse, four main spectral features were observed within the probe detection range. The photobleach (PB) negative signal centered around 2.86 eV (434 nm) was consistent with the lowest-energy feature observed in the steady-state absorption spectrum (Fig. 7b ). The second negative feature centered around 2.31 eV (537 nm) was also in good agreement with the central transition and lineshape of the measured PL spectrum (Fig. 7b ). Therefore, it was attributed to a stimulated emission (SE) process. Two positive signals associated with photoinduced absorption (PIA) processes were observed. The tail of the first one (PIA 1 ) was observed at the edge of the detection range, around 1.80 eV (689 nm); it was assigned to singlet-singlet transitions from VSs to higher-lying electronic states. The second positive signal (PIA 2 ) centered around 2.55 eV (486 nm) was assigned to transitions from CTS 1 to higher-lying states. Fig. 7a depicts the TA spectrum of MPC-1–2 , while Fig. 7b, c highlight the correlation between the main spectral features in the TA spectrum and their steady-state spectral counterparts. Fig. 7 Overview of transient absorption (TA) results and electronic model. a Pseudo-color map representing the TA spectra of MPC-1–2 . b Ultraviolet (UV)–visible (Vis) absorption (Abs) and PL spectra of MPC-1–2 . c Absorption difference spectral lines at various delays showing the position and evolution of the four features observed in the TA spectra. d Time constants of processes of interest extracted from fitting TA ( τ 1 – τ 3 ) and TRPL ( τ TRPL ) kinetics; CT VS2→CTS1 , CT VS1→CTS1 , PL VS2 , and PL VS1 indicate the` physical process associated with each time constant, respectively. Error bars represent the standard error at 1 σ . e Schematic of potential energy curves of the lowest electronic states of the heterodimer, D XY . Source data are provided as a Source Data file Full size image Four kinetic traces (one at each main spectral feature observed in the TA spectra) were extracted and fitted simultaneously with a sum of exponential functions employing a total of four time constants, τ 1 – τ 4 , (further information including details of the fitting model and procedure are presented in Supplementary Note 6 , Supplementary Fig. 9 , and Supplementary Table 12 ). Briefly, a sum of bi-exponential growth ( τ 1 , τ 2 ) and a single exponential decay ( τ 4 ) was utilized to simulate the PIA 2 kinetics, while a bi-exponential decay ( τ 2 , τ 3 ) was used to simulate both the PIA 1 and SE kinetics, which shared identical time constants. The slower time constant in PIA 2 ′s growth function ( τ 2 ) was shared with the fast decay component of PIA 1 /SE, while PB kinetic trace was simulated with a single exponential decay ( τ 4 ). Slow decay constants of PB and PIA 2 were also shared. Summary of relevant time constants are presented in Fig. 7d . The PIA 2 growth components ( τ 1 , τ 2 ) were assigned to relaxation to CTS 1 ; the faster component ( τ 1 < 5 ps) was assigned to the charge-transfer from VS 2 to CTS 1 (CT VS2→CTS1 ), while the slower component ( τ 2 < 20 ps) was assigned to the charge-transfer from VS 1 to CTS 1 (CT VS 1 →CTS1 ). This difference in observed time constants can be rationalized by the fact that the latter CT process is hindered by a barrier formed via the crossing of the VS 1 and CTS 1 potential energy surfaces (see Fig. 7e ). Furthermore, the slower growth component of PIA 1 ( τ 2 )  matches a detectable decay in SE and PIA 1 kinetics, both of which originate from the low-lying valance states, VS 1 and VS 2 . It is worth noting that the fast growth component ( τ 1 ) was not resolvable in either PIA 1 or SE signals in the TA measurement, likely due to their low signal-to-noise ratio. The slow decay component in PIA 1 and SE ( τ 3 ) was assigned to (radiative and non-radiative) decay processes originating from VS 2 (PL VS2 ). Time constant of the decay component of PIA 2 and PB ( τ 4 ) was deemed unreliable because its value is comparable with the time window of the TA apparatus (1.6 ns). Nevertheless, the estimated value of the time constant suggests a long lifetime of CTS 1 . Time-resolved photoluminescence (TRPL) measurements were carried out to deduce the lifetime of VS 1 (PL VS1 ), which was found to be about 10 ns for both MPC-1–1 and MPC-1–2 , consistent with the previously reported lifetimes of homopolymer PIM-1 and its isolated chromophore [54] . Further details and results of the TRPL data acquisition and analysis are presented in Supplementary Note 7 and Supplementary Figs. 10 and 11 . Combining experimental and computational results, the proposed photoinduced processes are described in Fig. 7e . The 3.2 eV (388 nm) pump laser excites the polymer to VS 1 and VS 2 . Facilitated by CIs, the charge-transfer process from VSs to CTS 1 occurs on a timescale of ≤ 20 ps. Relaxation of the bright VSs takes place in approximately 10 ns, while that of the dark CTS 1 is expected to be significantly longer. A photocatalytically active double-strand polymer system, MPC-1 , was developed and successfully employed in the hydrodehalogenation of α -halocarbonyl compounds in mostly excellent yields. Variation of the polymerization technique demonstrated the robustness of the substituent chromophores and led to the development of MPC-1–2 , an optimal preparation with improved catalytic activity and solubility properties. The recyclability of the photocatalyst was demonstrated in batch reactions, and a proof-of-concept flow cell reactor demonstrated the efficacy of the polymer when used as a transparent wall-coating. The backside irradiation approach employed in the flow reaction was found to be superior to use of the catalyst as a suspension and was effective even when the reaction mixture was made opaque with the addition of charcoal. Well-defined compounds were synthesized to clearly model the polymer substructure, and their catalytic activities supported the formation of beneficial CTSs within the model two-chromophore system. Steady-state absorption and PL spectra, as well as DFT calculations verified the Frenkel-Davydov exciton model in predicting the electronic structure of the polymer; features in the TA spectra can be well explained using this model. The recorded ultrafast kinetics supported the presence of long-lived CTS, which enable the polymer to act as an effective photocatalyst. General experimental details All manipulations were carried out under air unless otherwise noted. Solvent molarity listed in reaction schemes is relative to the limiting reagent. The molecular weight for all MPC-1 preparations ( MPC-1–0 , MPC-1–1 , MPC-1–2 , MPC-1–2 LMW , and MPC-1–2 HMW ) was approximated as 1529 g mol −1 , which corresponds to the constitutional unit of an ideal regular polymerization at the monomer ratio used in all preparations; the optimal polymer preparation, MPC-1–2 , was in very close agreement with this approximation based on NMR and GPC measurements. An analysis of the divergence of other preparations from this approximation is provided (see Supplementary Note 1 and Supplementary Figs. 12 – 17 ). All flash chromatography was conducted using a Teledyne Isco CombiFlash Rf 150. NMR spectra were recorded at 23 °C on Varian MR-400, Varian Unity INOVA 500, and Varian VNMRS 700 spectrometers (400, 500, and 700 MHz, respectively). Reported chemical shifts are referenced to residual solvent peaks. GCMS data was obtained using a Thermo Scientific Trace 1300 Gas Chromatograph coupled with a Thermo Scientific ISQ-QD Single Quadrupole Mass Spectrometer. Infrared absorbance spectra were acquired on a PerkinElmer Spectrum Two spectrometer using 1 cm −1 resolution unless stated otherwise. High-resolution mass analyses were obtained either using a 5975C Mass Selective Detector coupled with a 7890 A Gas Chromatograph (Agilent Technologies) or orbit-trap. Matrix-assisted laser desorption/ionization time-of-flight analyses were obtained using a Bruker Autoflex III. Supplies and chemicals Supplies : Thin-layer chromatography (TLC) plates (UV 254 indicator, aluminum backed, 175–225 µm thickness, standard grade silica gel, 230–400 mesh) were purchased from Merck. Silica gel (60 Å pore size, 230–400 mesh) was purchased from Silicycle. Sand was purchased from Fisher Chemical. Celite 545 was purchased from Acros Organics. Solvents : Acetone, ethyl acetate, hexanes, methanol, ethanol, N , N -dimethylformamide, dimethyl sulfoxide, dichloromethane, tetrahydrofuran, and high performance liquid chromatography (HPLC)-grade water were purchased from Fisher Chemical. Pentane, chloroform and 2-methyltetrahydrofuran were purchased from Sigma-Aldrich. N , N -Dimethylacetamide was purchased from Acros Organics. N -Methyl-2-pyrrolidone was purchased from Antec Inc. Acetonitrile was purchased from Pharmco Products Inc. 1,4-Dioxane was purchased from EMD Chemicals. NMR solvents were purchased from Cambridge Isotope Laboratories. Dry solvents were prepared using standard procedures [55] . Surfactant solutions were prepared in HPLC-grade water. PS-750-M (also known as FI-750-M) was prepared as previously reported [46] . TPGS-750-M and sodium dodecyl sulfate were supplied by Sigma-Aldrich. Substrates and reagents : 1,3,5-Trimethyl-1 H -pyrazole-4-sulfonyl chloride supplied by Maybridge was received as a gift from Novartis Pharmaceuticals. N , N -Diisopropylethylamine, sodium bicarbonate, and anhydrous potassium carbonate were purchased from Fisher Chemical. Diethyl 2,6-dimethyl-1,4-dihydropyridine-3,5-dicarboxylate (Hantzsch ester) was purchased from Combi-Blocks Inc. and Oakwood Chemicals, and both sources were confirmed to work equally well when adjusting loading based on NMR purity. 2,3,5,6-Tetrafluoroterephthalonitrile, 3,3,3′,3′-Tetramethyl-1,1′-spirobiindane-5,5′,6,6′-tetraol, 2-bromo-1-(4-bromophenyl)ethan-1-one, 1-([1,1′-biphenyl]-4-yl)-2-bromoethan-1-one, 2-bromo-1-(2-fluoro-5-methoxyphenyl)ethan-1-one, 1-(benzofuran-2-yl)-2-bromoethan-1-one, and 2-bromo-1-(3-bromo-4-fluorophenyl)ethan-1-one were purchased from Sigma-Aldrich. 2-Chloro-1-(2,4-dichlorophenyl)ethan-1-one and 2-bromo-1-(4-nitrophenyl)ethan-1-one were purchased from Oxchem Corporation and Oakwood Chemicals, and both sources were confirmed to work equally well. 2-Bromo-1,3-diphenylpropane-1,3-dione was purchased from Chem-Impex. (1 R ,3 S ,4 S )-3-Bromo-1,7,7-trimethylbicyclo[2.2.1]heptan-2-one was purchased from TCI. Sodium sulfinate, 2-bromo-1-(4-bromophenyl)propan-1-one, benzyl 2-bromoacetate and 1,2-dibromoethane were purchased from Acros Organics. 2-Chloro-1-(4-fluorophenyl)ethan-1-one, 2-bromo-2-methyl-1-phenylpropan-1-one, and tetrabutylammonium hexafluorophosphate were purchased from Oakwood Chemicals. 2,3,4,5,6-Pentafluorobenzonitrile was purchased from Matrix Scientific. 3-Bromo-1,3,4,5-tetrahydro-2 H -benzo[ b ]azepin-2-one was purchased from Ark Pharm. 2-Bromo-1-(2,4-dichlorophenyl)ethan-1-one and 1-(2,4-dichlorophenyl)-2-iodoethan-1-one were prepared by heating a 0.2 M dry acetone solution of 2-chloro-1-(2,4-dichlorophenyl)ethan-1-one at 70 °C in a thick-walled sealed reaction vessel with 1.5 equiv of sodium bromide and sodium iodide, respectively, and spectral data was in agreement with the literature [56] , [57] . 2,2-Dibromo-1-phenylethan-1-one was prepared as previously reported [58] . 2,3-Dibromo-2-methyl-3-phenylpropanal was prepared from 2,3-dibromo-2-methyl-3-phenylpropanal through the dropwise addition of 2 M bromine in dichloromethane (DCM) to a 0.2 M substrate in DCM solution at 0 °C followed by room temperature stirring and quenching with aqueous sodium sulfite, and spectral data was in agreement with the literature [59] . Preparation of polymer photocatalysts Polymer syntheses were partly adapted from published procedures [14] , [17] . Sulfone monomer 3 was prepared as described in Supplementary Method 2 . The MPC-1–0 catalyst was prepared as described in Supplementary Method 3 . NMR spectra are presented in Supplementary Figs. 18 – 26 . MPC-1–1 : Monomers 3 (1 equiv, 0.115 mmol), 1 (2 equiv, 0.23 mmol), and 2 (3 equiv, 0.345 mmol), and potassium carbonate (10 equiv, 1.15 mmol) were stirred at reflux in 4.6 mL 3 wt% PS-750-M for 2 h. The resultant yellow solid was collected over a fritted glass funnel by vacuum filtration and rinsed with deionized water. The solid was then suspended in 15 mL deionized water, stirred at reflux for 9 h, and again collected over a fritted glass funnel by vacuum filtration. After subjecting the solid to high vacuum for 2 h, it was dissolved in DCM and passed through a Celite plug. DCM was removed under reduced pressure, the solid was triturated in pentane. After removal of pentane, the solid was placed under high vacuum for 24 h. Greater detail and characterization is provided in Supplementary Method 4 . MPC-1–2 : Prior to use, monomer 1 (99%, Sigma-Aldrich) was sublimed under vacuum at 155 °C, monomer 2 (96%, Sigma-Aldrich) was recrystallized from methanol/water, and potassium carbonate (99.8%, Fisher Chemical) was dried overnight in an oven at 200 °C. A thick-walled Schlenk tube equipped with a polytetrafluoroethylene (PTFE)-coated stir-bar was charged with unactivated 3 Å molecular sieves (8–12 mesh, 400 mg) and potassium carbonate (9 equiv, 2.7 mmol) and then subjected to high vacuum at greater than 200 °C in a vacuum oven for 14 h. After cooling under vacuum, the vessel was removed and quickly charged with monomers 3 (1 equiv, 0.30 mmol), 1 (2 equiv, 0.60 mmol), and 2 (3 equiv, 0.90 mmol). The vessel was then briefly subjected to high vacuum and then backfilled with argon. With the vessel contents protected by positive argon pressure, dry DMAc was added by syringe. The vessel was subjected to magnetic stirring at 90 °C for 70 min, resulting in a viscous translucent yellow mixture. After cooling, the mixture congealed and 4 mL deionized water was added, resulting in a suspension of large yellow flakes. The vessel was sealed and magnetically stirred at 110 °C for 10 min and then at room temperature for 5 min. The supernatant liquid was removed by syringe and the yellow solid was thrice rinsed by stirring in 2 mL portions of deionized water, which were likewise removed. The yellow solid was then dissolved in 10 mL chloroform and admixed with 10 mL deionized water. The chloroform layer was transferred to a test tube, and the aqueous layer was extracted (2 × 1 mL chloroform). The combined chloroform layers were washed (1 × 1 mL deionized water) and then admixed with 10 mL methanol, causing the majority of the polymer to precipitate. The test tube was subjected to centrifugation, the supernatant liquid was decanted away, and the centrifuge pellet was dissolved in chloroform to transfer into a storage vial. Chloroform was removed under reduced pressure and the sample was placed under high vacuum at 130 °C for 16 h. Greater detail and characterization is provided in Supplementary Method 5 . Fractionations of MPC-1–2 : Twenty-eight milligrams of MPC-1–2 was dissolved in 1 mL chloroform and reprecipitated with 30 drops of methanol. The supernatant liquid was decanted. Precipitated solid was twice more reprecipitated from chloroform with methanol in the same manner. The solid thus obtained was designated as MPC-1–2 HMW . Solvent was removed from the combined supernatant layers under reduced pressure to give the fractionation designated as MPC-1–2 LMW . After the fractionations were subjected to high vacuum, they were obtained with approximately equal masses (14 mg). Optimization of hydrodehalogenation Detailed results from the optimization of the hydrodehalogenation reaction are provided in Supplementary Tables 2 – 9 . Except where otherwise noted, optimization reactions were conducted as follows. Solid reaction components were added to a spin-vane-equipped 10 × 75-mm borosilicate test tube that was then fitted with a 14/20 rubber septum. The septum was wrapped with PTFE tape, and the vessel was thrice evacuated and argon-backfilled. Liquid reaction components (including 1 equiv DMSO internal standard) were then added by syringe; the solvent (which had been sparged with argon for at least 10 min) was added last. The septum punctures were covered with electrical tape and the reaction vessel was placed in the photoreactor to stir under blue LED irradiation at 37 °C (see Supplementary Fig. 1 ). Samples for 1 H NMR monitoring of reaction progress were prepared by transferring a 20 µL reaction mixture aliquot into an empty NMR tube, quickly followed by the addition of 400 µL chloroform-d 6 and capping of the tube. Dehalogenation procedures Characterization of dehalogenation products is presented in Supplementary Note 8 , and NMR spectra are presented in Supplementary Figs. 27 – 46 . The photoreactor set-up is presented in Supplementary Fig. 1 . Solvents were not dried prior to use. Procedure A : The halide (1 equiv, 0.25 mmol) was added according to its phase at room temperature. Solid reaction components— MPC-1–1 (1 mol%), HE (1.5 equiv, 0.375 mmol), and halide (if solid)—were added to a spin-vane-equipped 10 × 75-mm borosilicate test tube that was then inserted into the narrow opening of a 14/20 rubber septum. The septum was wrapped with PTFE-tape, and the vessel was thrice evacuated/argon-backfilled. Halide (if liquid) and then 0.5 mL acetone (which had been sparged with argon for at least 10 min) were added by syringe. The septum punctures were covered with electrical tape, and the reaction vessel was placed in the photoreactor to stir under blue LED irradiation at 37 °C. Following reaction completion (as monitored by TLC or GCMS), the solvent was removed under reduced pressure, 0.5 mL deionized water was added, and the mixture was extracted with ethyl acetate (3 × 0.5 mL). The combined organic layers were dried over anhydrous magnesium sulfate, filtered, and concentrated under reduced pressure. The resultant crude residue was purified by flash chromatography. Procedure B : This method was employed for substrates that did not approach full conversion after 96 h with Procedure A. The halide (1 equiv, 0.25 mmol) was added according to its phase at room temperature. Solid reaction components— MPC-1–1 (2 mol%), the first portion of HE (1.5 equiv, 0.375 mmol), and halide (if solid)—were added to a spin-vane-equipped 10 × 75-mm borosilicate test tube that was then inserted into the narrow opening of a 14/20 rubber septum. The septum was wrapped with PTFE tape, and the vessel was thrice evacuated/argon-backfilled. Halide (if liquid) and then 1 mL acetone (which had been sparged with argon for at least 10 min) were added by syringe. The septum punctures were covered with electrical tape, the solvent level was marked on the outside of the vessel, and the vessel was placed in the photoreactor to stir under blue LED irradiation at 37 °C. Every 24 h, the reaction was monitored by TLC and GCMS, the solvent was replenished with sparged acetone to a slightly greater level than that of the initial volume, and the reaction mixture was directly sparged for several minutes. Following GCMS analysis at 72 h and prior to replenishing the solvent level, an additional 1 equiv HE was added under an argon cone, and the vessel was resealed and returned to the photoreactor. Workup and isolation were conducted as presented in Procedure A. Procedure C : The halide (1 equiv, 0.25 mmol), MPC-1–2 LMW (1 mol%), and HE (3 equiv, 0.75 mmol) were added to a spin-vane-equipped 10 × 75-mm borosilicate test tube that was then inserted into the narrow opening of a 14/20 rubber septum. The septum was wrapped with PTFE tape, and the vessel was thrice evacuated/argon-backfilled. A 1-mL volume of DMSO (which had been sparged with argon for at least 10 min) was added by syringe. The septum punctures were covered with electrical tape, and the reaction vessel was placed in the photoreactor to stir under blue LED irradiation at 37 °C. The reaction was monitored for completion by TLC. Following reaction completion, the reaction mixture was transferred to a 16 × 100-mm test tube, 1 mL ice-cold deionized water was added, and the mixture was extracted with ethyl acetate (3 × 1 mL). The combined organic layers were dried over anhydrous magnesium sulfate, filtered, and concentrated under reduced pressure. The resultant crude residue was purified by flash chromatography. Gram-scale hydrodehalogenation : Halide 4b (1 equiv, 5.0 mmol, 1176 mg), MPC-1–1 (0.2 mol%, 15 mg), and the first portion of HE (1.1 equiv, 5.5 mmol, 1436 mg), were added to a stir-bar-equipped 25-cm 3 round-bottom flask, which was then fitted with a rubber septum. The septum was wrapped with PTFE tape, and the vessel was thrice evacuated/argon-backfilled. A 10-mL volume of acetone (which had been sparged with argon for 10 min) was added by syringe. The septum punctures were covered with electrical tape, and the reaction vessel was placed in the photoreactor to stir under blue LED irradiation at 37 °C. Reaction monitoring at 15 h by 1 H NMR showed ca. 60% conversion to product 5b and also indicated that the first HE portion had been exhausted. At 16 h, the second portion of HE (0.9 equiv, 4.5 mmol, 1175 mg) was added while briefly opening the vessel under an argon cone. At 24 h, the vessel was removed from the photoreactor and acetone was removed under reduced pressure. Extractions were conducted by admixing ethyl acetate to solubilize the polymeric residue and then admixing a 9–14 times larger volume of hexanes to reform the polymeric phase. Supernatant organic layers were combined, solvent was removed under reduced pressure, and the crude reaction mixture was purified by flash chromatography (ethyl acetate/hexanes), affording product 5b in 99% isolated yield (936 mg clear faintly yellow oil), as confirmed by 1 H NMR. Electron microscopy SEM was conducted with a TESCAN Vega3 SEM. HRTEM was conducted with a 200-kV FEI Tecnai F20 FEG-TEM/STEM. Additional SEM and HRTEM images are provided in Supplementary Figs. 47 and 48 . Gel-permeation chromatography GPC was conducted on an Omnisec GPC from Malvern equipped with four on-line detectors: a dual-angle light scattering detector, a refractive index detector, a UV detector, and a viscosity detector. Samples were fully dissolved in THF and eluted through two columns (Viscotek, LT5000L and LT 3000L) at a rate of 1 mL min −1 . MPC-1–0 was not fully soluble in THF and was not analyzed. More detailed results are provided in Supplementary Figs. 49 – 54 . Estimation of the average number of chromophores in different MPC-1 preparations is presented in Supplementary Note 9 and Supplementary Tables 13 – 16 . Benchmarking studies Reaction vessels were prepared using halide 4b according to Procedure A (except with different catalysts) unless otherwise noted. The molecular weight for MPC-1 preparations was approximated as 1529 g mol −1 , based on the constitutional unit of an ideal regular polymerization; this constitutional unit contained three chromophores (two terephthalonitrile units and one sulfone unit). The loading for other catalysts was adjusted so as to keep the number of active units constant. Accordingly, the catalyst loading was 3 mol% with respect to active catalytic units. After stirring for 2 h under blue LED irradiation, mesitylene was added by microsyringe, and the reaction mixture was agitated to uniformly incorporate the internal standard. A 20 µL aliquot was then withdrawn by syringe and transferred to an empty NMR tube, quickly followed by the addition of 400 µL chloroform-d 6 and capping of the tube. A combined set of benchmarking results is presented in Supplementary Table 17 . Recycle studies Details for the recycle study with MPC-1–1 are provided in Supplementary Method 1 . The recycle study with polymeric MPC-1–2 LMW (Fig. 3a ) was conducted using halide 4b and Procedure A (except that the catalyst and workup were changed) for the zeroth cycle (Fig. 3a ). Each recycle: additional halide 4b (1 equiv, 0.25 mmol) and HE (1.5 equiv, 0.375 mmol) were added to the recovered MPC-1–2 LMW catalyst (1 mol%, 3.8 mg) originating from the zeroth cycle; the reaction vessel was septum/PTFE-tape-sealed, thrice evacuted/argon-backfilled, and then filled with 0.5 mL argon-sparged acetone; the punctures were sealed with electrical tape, and the reaction vessel was placed in the photoreactor to stir under blue LED irradiation at 37 °C. For each cycle: after 3 h in the photoreactor, the vessel was removed from irradiation and its contents were diluted with 0.5 mL methanol; the resultant suspension was then passed through a fritted glass funnel, rinsing with additional methanol; the recovered solid catalyst was returned to the reaction vessel; the filtrate solvent was removed under reduced pressure, and the resultant crude residue was purified by flash chromatography (ethyl acetate/hexanes) to provide product 5b as a clear slightly yellow oil. Product purity was confirmed by 1 H NMR. The catalyst was typically returned to the reaction vessel by passing it through the frit with DCM, which was subsequently removed under reduced pressure, but after the third recycle the catalyst was returned to the reaction vessel as a solid using a spatula, and no deterioration in activity was observed. Flow reactor study The set-up for the flow reactor is pictured in Fig. 3b and Supplementary Fig. 55 . MPC-1–2 HMW (2.5 mol%, 26.5 mg) was dissolved in a minimal volume of DCM and transferred into a glass flow cell. Keeping the path through the cell parallel to the ground, the cell was rotated so as to coat the walls as the DCM evaporated. Small portions of DCM were added to the cell to reapply any portions of the film, which formed without adhering to the glass. Once the catalyst was evenly coated on the flow cell walls, the vessel was subjected to rotary evaporation and then high vacuum for 2 h. Halide 4b (1 equiv, 0.700 mmol) was placed in a conical microwave vial, and HE (1.5 equiv, 1.05 mmol) was added to the MPC-1–2 HMW -coated flow cell. The microwave vial was fitted with a septum that had been punctured to allow two pieces of PTFE tubing to be threaded into the vessel. The other two ends of PTFE tubing pieces were connected to the flow cell, and the entire apparatus was thrice evacuated/argon-backfilled before adding 3.5 mL of argon-sparged acetonitrile to the microwave vial reservoir and placing an argon balloon needle into its septum. The reservoir was swirled until the halide completely dissolved, and then one of the pieces of PTFE tubing was attached to a peristaltic pump near the photoreactor. The reactor cell was suspended in the photoreactor horizontally so as to allow the bed of HE to sit evenly across the bottom of the flow cell. Within the microwave vial, one piece of PTFE tubing was inserted all the way to the bottom of the solution while the other was kept close to the top of the vessel. The microwave vial was covered with aluminum foil to exclude the possibility of irradiation of the reservoir having any impact on the reaction. Peristaltic pumping was initiated, and the reaction was monitored by GCMS. After 26 h, the reaction was stopped, and the flow loop was drained by lifting the PTFE tubing above the reservoir liquid level. The flow loop was subsequently rinsed with 2.0 mL acetonitrile. The solvent in the reservoir was removed under reduced pressure and the product was isolated by flash chromatography in 83% yield, as confirmed by NMR. Cyclic voltammetry Cyclic voltammetry measurements were conducted with a Gamry Interface 1000 potentiostat using a glassy carbon working electrode (0.071 cm 2 surface area), a platinum wire counter electrode, and a silver wire pseudo-reference electrode. Prior to use, the working electrode was polished with aqueous alumina slurry, and both the working and counter electrodes were cleaned by washing sequentially with water, ethanol, acetone, and dichloromethane and then sonicating in dichloromethane for 15 min. A three-neck electrochemical cell was washed and oven-dried prior to use. Measurements were taken at a scan rate of 200 mV s −1 under a nitrogen atmosphere using a 25 mL volume of 0.1 M ( n- Bu) 4 NPF 6 in dichloromethane. Potentials were referenced to ferrocene and adjusted to be presented relative to SCE by adding 0.380 V. In the presence of the supporting electrolyte, MPC-1–2 exhibited limited solubility. Voltammograms were obtained for the solvent blank, and after each sequential addition of MPC-1–2 , ferrocene, halide 4b , and Hantzsch ester to the electrochemical cell (Supplementary Fig. 56 ). Preparation of polymer subunit models All polymer subunit models were prepared as mixtures of isomers; for simplicity, only one product structure is depicted and named in each case. Detailed synthetic procedures and product characterization are provided in Supplementary Methods 6 – 12 , and NMR spectra are presented in Supplementary Figs. 57 – 73 . Charcoal occlusion study Four 10 × 75-mm borosilicate test tubes were etched with a diamond Dremel bit so that etches were not more than ca. 1 mm apart and covered at least the bottom 25 mm of the tubes. Catalyst was delivered to all tubes as equal volumes of DCM-dissolved MPC-1–2 HMW . Two of the vessels were deignated to use the catalyst as a coating, and for these vessels the DCM was removed by evaporation, then a minimal amount of DCM was added to spin coat the catalyst such that it covered the bottom 25 mm of the tubes; after spin coating, these vessels were subjected to rotary evaporation and high vacuum, and then two 0.5 mL hexanes rinses were added and removed under reduced pressure. The other two vessels were designated to use the catalyst as a suspension, and for these vessels 0.5 mL hexanes was added to the DCM to precipitate the polymer, and then the solvent was removed by rotary evaporation; an additional 0.5 mL hexanes was added and the polymer precipitate was triturated before removing the hexanes by rotary evaporation. All four vessels were then subjected to high vacuum for 2 h. To each vessel was added a spin-vane (pointed end up), halide 4b (1 equiv, 0.2 mmol), and Hantzsch ester (1.5 equiv, 0.3 mmol). For one vessel using the catalyst as a coating and one vessel using the catalyst as a suspension, 4 mg activated charcoal was added. Vessels were then septum-sealed, thrice evacuated/argon-backfilled, and then filled with 1 mL acetonitrile (which had been sparged with argon for 1 h). Punctures were covered with electrical tape and septa were wrapped with PTFE tape before placing the vessels in the photoreactor, and the stir plate was adjusted to stir just fast enough for the charcoal to be evenly dispersed throughout the reaction vessels. Reactions were periodically monitored by NMR analysis of 20 µL aliquots. Immediately prior to the first monitoring, mesitylene internal standard was admixed. Tabulated results are provided in Supplementary Table 18 . Steady-state absorption and photoluminescence studies Steady-state absorption measurements were carried out on a Cary Bio 50 UV–Vis spectrometer (Agilent Technologies), in a sealed quartz cuvette with a 1-mm optical path length. Samples were dissolved in chloroform and purged with nitrogen for 30 min prior to measurement. Absorption was collected from 1.77 to 6.2 eV (200 to 700 nm). Ten separate scans of the same sample were acquired and averaged. A chloroform absorption spectrum was collected and subtracted from the spectra of all solutions. PL measurements were conducted using an LS 55 fluorescence spectrometer (PerkinElmer) with a sealed quartz cuvette with a 10-mm optical path length. Samples were dissolved in chloroform and purged with nitrogen for 30 min prior to measurement. Three excitation energies were explored: 4.2 eV (295 nm), 3.1 eV (400 nm), and 2.8 eV (445 nm). Emission was collected from 1.8 to 2.95 eV (690 to 420 nm). PL spectra were associated with singlet transitions (Supplementary Note 10 and Supplementary Fig. 74 ). Femtosecond transient absorption spectroscopy studies TA data of the samples was acquired from solutions in chloroform. Sample concentration was adjusted so that the approximate concentration of chromophore units per unit volume was ~150 µM. Sample solutions were purged with nitrogen gas for 30 min, and the measurements were carried out in a sealed quartz cuvette with a 1-mm optical path length. The pump-probe experimental set-up employed to acquire the TA data presented in this work utilizes a Clark-MXR ShapeShifter, a Ti:sapphire mode-locked regenerative amplifier laser system (Clark-MXR, CPA, wavelength = 775 nm, pulse duration ≲ 150 fs, pulse energy ∼ 1 mJ at 1 kHz repetition rate). Details of the experimental set-up are explained elsewhere [60] , [61] , [62] . To improve the signal-to-noise ratio, and maintain a consistent time profile, ten individual delay scans were carried out on each sample, each of which was averaged over 500 pulses per delay step, and then all ten scans were averaged. Pump fluence was maintained around 250 µJ cm −2 during all the scans. Using the same overlap and fluence characteristics, the cuvette filled with chloroform was measured five times within the first 5 ps delay, and the average of those measurements was subtracted from the average of the sample measurement within that delay window. Group velocity desperation was corrected by applying a 3rd-order polynomial to the Time–Wavelength axes. Delay time steps were distributed linearly between −1 and 1 ps, with 20 fs steps, and logarithmically after 1 ps such that each order of magnitude contained 100 steps. Reporting summary Further information on experimental design is available in the Nature Research Reporting Summary linked to this article.